The translation inhibitor pateamine A prevents cachexia-induced muscle wasting in mice Cachexia, or muscle-wasting syndrome, is one of the major causes of death in patients affected by diseases such as cancer, AIDS and sepsis. However, no effective anti-cachectic treatment is currently available. Here we show that a low dose of pateamine A, an inhibitor of translation initiation, prevents muscle wasting caused by the cytokines interferon γ and tumour necrosis factor α or by C26-adenocarcinoma tumours. Surprisingly, although high doses of pateamine A abrogate general translation, low doses selectively inhibit the expression of pro-cachectic factors such as inducible nitric oxide synthase. This selectivity depends on the 5′UTR of inducible nitric oxide synthase messenger RNA (mRNA) that, unlike the 5′UTR of MyoD mRNA, promotes the recruitment of inducible nitric oxide synthase mRNA to stress granules, where its translation is repressed. Collectively, our data provide a proof of principle that nontoxic doses of compounds such as pateamine A could be used as novel drugs to combat cachexia-induced muscle wasting. Cachexia, characterized by excessive weight loss and skeletal muscle deterioration (muscle wasting), is a disorder that often affects individuals with cancer, AIDS, chronic obstructive pulmonary disease and sepsis [1] , [2] . These individuals lose skeletal muscle mass owing to a decreased rate of synthesis and enhanced degradation of muscle proteins. Cancer patients affected by cachexia experience a lower quality of life and respond more poorly to therapy, and ~30% of all cancer-related deaths are the direct result of cachexia-induced muscle wasting [1] , [2] . Despite the fact that Cachexia and its consequences have been known for decades, there are no effective treatments to prevent its onset and/or progression. Although the symptoms of cachexia are diverse, several key mediators have been identified. Pro-inflammatory cytokines, such as interferon γ (IFNγ) and tumour necrosis factor α (TNFα), have been shown to induce muscle wasting in individuals affected with cancer or chronic inflammation [3] , [4] , [5] . The ability of both IFNγ and TNFα to induce muscle wasting is mediated by the activation of the transcription factor NF-κB [5] , [6] . One of the main consequences of activating the NF-κB pathway in muscle fibres is the decreased expression of key factors required for the formation and maintenance of muscle fibres such as MyoD, Myogenin and the myosin heavy chain (MyHC) [5] , [6] , [7] . Furthermore, induction of the NF-κB pathway enhances the expression of the E3 ligase MURF1, which, in turn, activates the ubiquitin-proteasome pathway resulting in the degradation of proteins during muscle wasting [8] , [9] . One of the principal effectors of NF-κB-mediated muscle wasting is nitric oxide (NO), a gas normally secreted by cells to defend against pathogenic infections [2] , [6] , [10] . NO is produced as a result of the conversion of L -arginine to citrulline by enzymes such as inducible NO Synthase (iNOS) [11] . NO mediates several of the deleterious consequences associated with an aggravated pro-inflammatory response, including cytokine-induced muscle wasting [1] , [6] , [12] . Indeed, treatment of muscle cells with IFNγ and TNFα stimulates, in an NF-κB-dependent manner, the expression of iNOS and, subsequently, the secretion of NO [6] , [10] . The importance of NO in muscle wasting was demonstrated in vivo using an iNOS inhibitor, which prevented the onset of muscle loss and the subsequent death of animals that occurred on induction of cachexia [13] . Moreover, the NF-κB-induced decrease in MyoD messenger RNA levels in muscle fibres is mediated by the iNOS/NO pathway [6] . These results, therefore, suggest that targeting the iNOS/NO pathway could prove to be an effective treatment option to prevent cachexia-induced muscle wasting. Compounds known to inhibit eukaryotic initiation of translation possess anti-tumorigenic and immunosuppressive properties [14] , [15] . Recently, compounds such as Pateamine A (PatA, isolated from the marine sponge Mycale sp .) and silvestrol (an isomer of Episilvestrol (Epi), isolated from the genus Aglaia ) were found to mediate these effects by specifically altering the activity of eIF4A (a component of the eIF4F complex needed for the assembly of the 40 s ribosome subunit) [16] , [17] , [18] , [19] , [20] , [21] . Several studies have demonstrated that this family of small molecules preferentially inhibits the expression of messages that mediate the onset of certain diseases by acting on their 5′ untranslated regions (5′UTRs) [16] , [22] . In addition, PatA also mediates translation inhibition by inducing the formation of stress granules (SGs), cytoplasmic foci, that assemble in response to a variety of stresses [23] , [24] . On assembly, SGs recruit stalled translation pre-initiation complexes, along with RNA-binding proteins such as eIF4A, FXR1 (Fragile X mental retardation syndrome-related protein) and HuR (Human antigen R) [24] , [25] , [26] , [27] . Selective recruitment of specific mRNA transcripts into SGs leads to their increased stability and translational inhibition [26] , [28] , [29] , [30] . As tumours and inflammation are conditions that lead to muscle wasting, we tested the use of the translation initiation inhibitors PatA and Epi as potential anti-cachectic agents. As a proof of principle, we assessed the effect of different doses of PatA on TNFα/IFNγ- and tumour-induced muscle wasting. We observed that a low dose of PatA blocks the onset of muscle wasting both in vitro and in vivo. This effect is mediated by a novel and unexpected mechanism through which PatA, while inhibiting iNOS mRNA translation in a 5′UTR-dependent manner, promotes the expression of MyoD and Myogenin. Our result also show that the inhibition of iNOS translation by PatA is likely due to an increased association of its mRNA to eIF4A and the accumulation of iNOS mRNA/eIF4A complex in SGs. Our data suggest that these small molecules could be used as a novel strategy to combat the onset and progression of cachexia. Pateamine A blocks cytokine-induced muscle wasting PatA prevents, in a dose-dependent manner, the proliferation of cancer cells by inhibiting DNA synthesis during the S phase of the cell cycle [31] . Because myogenesis (the process of muscle fibre formation) requires the cell cycle arrest of myoblasts (embryonic muscle cells) [32] , we verified the effect of PatA on this process. C2C12, an established muscle cell line [33] , was induced to differentiate for 4 days in the presence or absence of different doses of PatA. Whereas doses of PatA >0.025 μM induced the death of undifferentiated myoblasts, lower doses enhanced the efficiency of muscle cell differentiation ( Fig. 1a ). These results were confirmed when the expression of MyHC and myoglobin, two bona fide markers of muscle cell differentiation [32] , was assessed by immunofluorescence ( Fig. 1b ). We observed that 0.0125 μM PatA promoted muscle differentiation, as indicated by the significant increase in the fusion index of differentiated myofibres [32] ( Fig. 1c ). Western blot analysis supported these results and showed that PatA, but not 100 μM aminoguanidine (AMG) (a specific inhibitor of the iNOS protein [6] ), significantly increased the expression of MyHC ( Fig. 1d,e ). These observations show that a low dose of PatA promotes muscle fibre formation when added during the early steps of the process. However, when we repeated similar experiments on fully formed myofibres we observed that, unlike undifferentiated muscle cells, they tolerated higher doses of PatA. Concentrations of PatA of 0.25 μM or more triggered the loss of myofibres ( Fig. 1f ), as indicated by the activation of apoptosis (assessed by determining the percentage of apoptotic nuclei and by the activation of caspase-3 cleavage [34] ) ( Fig. 1g,h ) and the complete inhibition of general translation ( Fig. 1i,j ). However, doses of 0.1 μM PatA or lower had no effect on the integrity of fully formed myofibres ( Fig. 1f–j ). 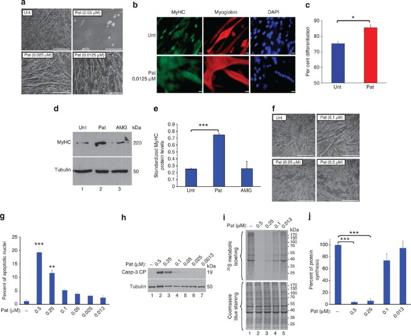Figure 1: Low doses of PatA are not detrimental to muscle fibres (a–e). Low doses of PatA promote myogenesis. (a) Phase-contrast images of myofibres that were treated during the differentiation process with or without the indicated concentrations of PatA for 96 h. Images are representative of three independent experiments. Bars, 50 μM. (b) Myotubes formed in the presence or absence of 0.0125 μM PatA were used for immunofluorescence analysis with anti-myoglobin and anti-MyHC antibodies. Bars, 20 μm. (c) Graph depicting the fusion index of muscle fibres seen in b from at least three fields from three independent experiments±s.e.m. *P<0.05 (Student'st-test). (d) Western blot analysis of MyHC protein levels in myofibres treated with or without 0.0125 μM PatA or 100 μM AMG. Tubulin protein levels are included as a loading control. (e) The MyHC levels in the western blot (d) were quantified, normalized against Tubulin protein levels and plotted±s.e.m. from three independent experiments. ***P<0.001 (Student'st-test). (f–h) Low doses of PatA do not affect the integrity of muscle fibres. (f) Phase-contrast images of myofibres assessed 24 h post-treatment with different doses of PatA. Images are representative of three independent experiments. Bars, 50 μm. (g) Myofibres were stained with DAPI to visualize apoptotic nuclei. Values are presented as percentages±s.e.m. of three independent experiments. **P<0.01, ***P<0.001 (Student'st-test). (h) Western blot analysis of caspase 3 cleavage product (indicative of apoptosis) in myofibres treated with different doses of PatA. Tubulin protein levels were included as a loading control. Immunoblots are representative of three independent experiments. (i,j) PatA inhibits protein synthesis in a dose-dependent manner. Myofibres treated with different concentrations of PatA were assessed forde novoprotein synthesis. (i) Thede novosynthesis of protein was detected by autoradiography (top panel). Coomassie blue staining of gels were performed to assess total protein levels (lower panel). (j) The effect of PatA on protein synthesis detected by autoradiography was standardized (using the total protein content obtained from Coomassie blue staining) and plotted as a percentage±the s.e.m. from four independent experiments. ***P<0.001 (Student'st-test). Figure 1: Low doses of PatA are not detrimental to muscle fibres ( a – e ). Low doses of PatA promote myogenesis. ( a ) Phase-contrast images of myofibres that were treated during the differentiation process with or without the indicated concentrations of PatA for 96 h. Images are representative of three independent experiments. Bars, 50 μM. ( b ) Myotubes formed in the presence or absence of 0.0125 μM PatA were used for immunofluorescence analysis with anti-myoglobin and anti-MyHC antibodies. Bars, 20 μm. ( c ) Graph depicting the fusion index of muscle fibres seen in b from at least three fields from three independent experiments±s.e.m. * P <0.05 (Student's t -test). ( d ) Western blot analysis of MyHC protein levels in myofibres treated with or without 0.0125 μM PatA or 100 μM AMG. Tubulin protein levels are included as a loading control. ( e ) The MyHC levels in the western blot ( d ) were quantified, normalized against Tubulin protein levels and plotted±s.e.m. from three independent experiments. *** P <0.001 (Student's t -test). ( f–h ) Low doses of PatA do not affect the integrity of muscle fibres. ( f ) Phase-contrast images of myofibres assessed 24 h post-treatment with different doses of PatA. Images are representative of three independent experiments. Bars, 50 μm. ( g ) Myofibres were stained with DAPI to visualize apoptotic nuclei. Values are presented as percentages±s.e.m. of three independent experiments. ** P <0.01, *** P <0.001 (Student's t -test). ( h ) Western blot analysis of caspase 3 cleavage product (indicative of apoptosis) in myofibres treated with different doses of PatA. Tubulin protein levels were included as a loading control. Immunoblots are representative of three independent experiments. ( i,j ) PatA inhibits protein synthesis in a dose-dependent manner. Myofibres treated with different concentrations of PatA were assessed for de novo protein synthesis. ( i ) The de novo synthesis of protein was detected by autoradiography (top panel). Coomassie blue staining of gels were performed to assess total protein levels (lower panel). ( j ) The effect of PatA on protein synthesis detected by autoradiography was standardized (using the total protein content obtained from Coomassie blue staining) and plotted as a percentage±the s.e.m. from four independent experiments. *** P <0.001 (Student's t -test). Full size image As one of the main characteristics of cachexia is a reduction in the levels of promyogenic factors, such as MyHC and Myogenin [1] , [5] , [6] , [35] , we tested whether PatA could reverse these outcomes. One of the well-established models that mimics cachexia in vitro is the treatment of myofibres with IFNγ and TNFα [5] , [6] , [35] . We observed that 0.1 μM PatA prevented the loss of fully differentiated C2C12 myofibres that is normally seen after treatment with IFNγ (100 U ml −1 ) and TNFα 20ng ml −1 ) for 72–96 h ( Fig. 2a ). In addition, immunofluorescence experiments showed that although IFNγ/TNFα led to a reduction in the number (>35%) and size (>45%) of myofibres exposed to these two cytokines, these effects were reversed in the presence of 0.1μM PatA ( Fig. 2b–d ). Likewise, the expression of the MyHC and Myogenin proteins (as determined by western blot analysis) were significantly greater when 0.1 μM PatA was added to myofibres in the presence of IFNγ/TNFα compared with myofibres treated with these two cytokines alone ( Fig. 2e–g ). Epi, an isomer of silvestrol that impacts eIF4A activity similarly to PatA [16] , also prevented the onset of IFNγ/TNFα-induced muscle wasting ( Supplementary Fig. S1a,b ). These observations suggest that when used at a low dose, compounds such as PatA and Epi prevent muscle wasting. 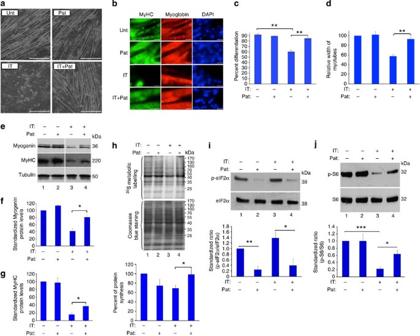Figure 2: PatA prevents IFNγ/TNFα-induced muscle wasting. (a–g) Effect of PatA on myofibres exposed to cytokines. (a) Phase-contrast images demonstrating the effect of 0.1 μM PatA on myofibres treated with or without IFNγ (100 U ml−1) and TNFα (20 ng ml−1) for 72–96 h. Bars, 50 μm. Images are representative of four independent experiments. (b) Myotubes treated with or without IFNγ (100U ml−1) and TNFα (20 ng ml−1) in the presence or absence of 0.1 μM PatA were used for immunofluorescence analysis with anti-myoglobin and MyHC antibodies. Bars, 20 μm. (c) Graph depicting the fusion index of muscle fibres seen in (b) from at least three fields from three independent experiments±s.e.m. **P<0.01 (Student'st-test). (d) The mean diameter of the fibres seen in (b) (see white lines in panels for examples of diameters measured) was determined and represented on the graph as a percentage relative to the diameter of untreated myofibres±s.e.m. of three independent experiments. **P<0.01 (Student'st-test). (e) Western blot analysis of Myogenin and MyHC protein levels in myofibres treated with or without 0.1 μM Pat in the presence or absence of IFNγ/TNFα. (f,g) The Myogenin or MyHC protein levels, described above, were quantified using ImageQuant, normalized against the loading control and plotted±the s.e.m. from three independent experiments. *P<0.05 (Student'st-test). (h–j) PatA rescues the decrease in protein synthesis that occurs in IFNγ/TNFα-treated C2C12 muscle fibres. (h)De novoprotein synthesis was determined as described inFig. 1i–jby plotting the average percentage values±the s.e.m. from four independent experiments. *P<0.05 (Student'st-test). (i,j) Western blot analysis of phospho-eIF2α (i, top panel) and phospho-S6 (j, top panel) levels in myofibres collected 24 h after treatment with or without 0.1 μM PatA in the presence or absence of IFNγ/TNFα. Total eIF2α and S6levels were used as a loading control. The phospho-eIF2α and phospho-S6levels were quantified, normalized against eIF2α level and S6 level, respectively, and plotted±the s.e.m. from 3 independent experiments (bottom panels). *P<0.05, **P<0.01, ***P<0.001 (Student'st-test). Figure 2: PatA prevents IFNγ/TNFα-induced muscle wasting. ( a–g ) Effect of PatA on myofibres exposed to cytokines. ( a ) Phase-contrast images demonstrating the effect of 0.1 μM PatA on myofibres treated with or without IFNγ (100 U ml −1 ) and TNFα (20 ng ml −1 ) for 72–96 h. Bars, 50 μm. Images are representative of four independent experiments. ( b ) Myotubes treated with or without IFNγ (100U ml −1 ) and TNFα (20 ng ml −1 ) in the presence or absence of 0.1 μM PatA were used for immunofluorescence analysis with anti-myoglobin and MyHC antibodies. Bars, 20 μm. ( c ) Graph depicting the fusion index of muscle fibres seen in ( b ) from at least three fields from three independent experiments±s.e.m. ** P <0.01 (Student's t -test). ( d ) The mean diameter of the fibres seen in ( b ) (see white lines in panels for examples of diameters measured) was determined and represented on the graph as a percentage relative to the diameter of untreated myofibres±s.e.m. of three independent experiments. ** P <0.01 (Student's t -test). ( e ) Western blot analysis of Myogenin and MyHC protein levels in myofibres treated with or without 0.1 μM Pat in the presence or absence of IFNγ/TNFα. ( f,g ) The Myogenin or MyHC protein levels, described above, were quantified using ImageQuant, normalized against the loading control and plotted±the s.e.m. from three independent experiments. * P <0.05 (Student's t -test). ( h–j ) PatA rescues the decrease in protein synthesis that occurs in IFNγ/TNFα-treated C2C12 muscle fibres. ( h ) De novo protein synthesis was determined as described in Fig. 1i–j by plotting the average percentage values±the s.e.m. from four independent experiments. * P <0.05 (Student's t -test). ( i,j ) Western blot analysis of phospho-eIF2α ( i , top panel) and phospho-S6 ( j , top panel) levels in myofibres collected 24 h after treatment with or without 0.1 μM PatA in the presence or absence of IFNγ/TNFα. Total eIF2α and S6levels were used as a loading control. The phospho-eIF2α and phospho-S6levels were quantified, normalized against eIF2α level and S6 level, respectively, and plotted±the s.e.m. from 3 independent experiments (bottom panels). * P <0.05, ** P <0.01, *** P <0.001 (Student's t -test). Full size image PatA and Epi belong to a family of natural molecules that, at relatively high doses, inhibit general translation [16] , [19] , [36] . As one of the main features of muscle wasting is a rapid decrease in protein synthesis [1] , the results described above raise the interesting and unexpected possibility that, at low doses, these compounds could prevent muscle loss by reestablishing general translation. 35 S-Meth in vivo labelling experiments [29] showed that 0.1 μM PatA reversed the 30% inhibition of general translation observed in myofibres treated with IFNγ/TNFα alone ( Fig. 2h ). This effect of PatA was accompanied by the simultaneous dephoshorylation of the translation initiation factor eIF2α and the phosphorylation of the S6 protein, a known target of the mTOR pathway ( Fig. 2i,j ). Given that the decrease in protein synthesis observed during muscle wasting is linked to eIF2α phosphorylation and S6 dephosphorylation [1] , [37] , [38] , our data demonstrate that a low dose of PatA prevents muscle loss, at least in part, by reestablishing general translation. PatA prevents muscle wasting in vivo We next assessed whether PatA can prevent cachexia in vivo . The injection of C26 adenocarcinoma cells in BALB/C mice induces the formation of tumours that causes muscle wasting in IL-6-dependent manner [35] , [39] , [40] . Consistent with these observations, our data show that the C26-induced tumours trigger a loss of body weight and muscle mass, a decrease in the expression levels of the MyoD mRNA, as well as an increase in the level of iNOS expression ( Supplementary Fig. S2 ). To test the effect of PatA in this system, we injected BALB/C mice with C26 cells, and 6 days later, these mice were treated with or without 50 μg kg −1 PatA and every second day thereafter, until day 19. While, as expected [31] , this treatment significantly reduced the size and weight of the C26-tumours, it also prevented the C26-induced wasting of the gastrocnemius muscle ( Supplementary Fig. S3a–e ). To determine whether PatA could prevent muscle wasting without affecting tumour growth, we used a lower dose of PatA (20 μg kg −1 ). We found that although this dose of PatA has no effect on body weight nor caused any significant signs of distress in mice ( Supplementary Fig. S3f ), it prevented the C26-induced muscle loss without having a significant effect on the volume and mass of the tumour itself ( Fig. 3a–e ). 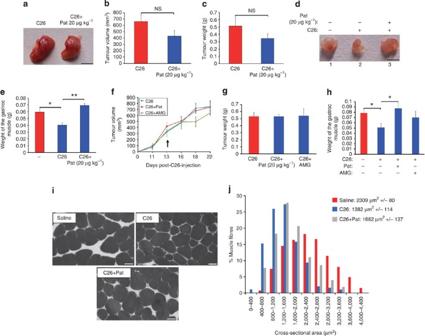Figure 3: PatA suppresses tumour-induced muscle wasting in BALB/c mice injected with C26 adenocarcinoma cells. (a–e) Injection of mice with 20 μg kg−1PatA 6 days post-injection of C26 adenocarinoma cells prevents muscle wasting without affecting tumour growth. Mice were treated with or without 20 μg kg−1of PatA starting at 6 days post-injection of C26 cells and every second day thereafter. Mice were subsequently killed 19 days after the injection of C26 cells. (a) Photographs of the tumours are representative ofn=3 mice per sample group. Bars, 5 mm. Tumour volume (b) and weight (c)±s.e.m. were measured for 3 mice per group. NS refers to non-significance. (d) Photograph and (e) weight of gastrocnemius muscles isolated from mice described above. Photographs indare representative ofn=3 mice, Bars, 5 mm. Weights ineare presented±s.e.m. fromn=3 mice per group. *P<0.05, **P<0.01 (Student'st-test). (f–j) Injection of 20 μg kg−1PatA in C26 tumour-bearing mice prevents muscle atrophy. (f) Effect of 20 μg kg−1PatA or 50 mg kg−1AMG on the growth of C26 tumours. Tumour volumes were calculated over a 3-week period. PatA or AMG was only injected into mice on day 13 (indicated on graph by a black arrow) when tumours became palpable and every second day thereafter. The mice were killed on day 22 after the injection of C26 cells. Volumes are presented as ±s.e.m. fromn=3 mice. (g) Weight of tumours and (h) gastrocnemius muscles isolated from mice 22 days post-C26 injection treated or not with 20 μg kg−1of PatA or 50 mg kg−1AMG, as described above. Weights are presented ±s.e.m. fromn=3 mice per group. (h) *P<0.05 (Student'st-test). (i) Immunohistochemical staining of gastrocnemius muscle fibres isolated from saline as well as C26 tumour-bearing mice treated with or without PatA, as described above. Bars, 20 μm. (j) The cross-sectional area of muscle fibres described iniare represented as a frequency histogram fromn=2 mice. The mean cross-sectional area of the fibres is indicated in the histogram±s.e.m. Figure 3: PatA suppresses tumour-induced muscle wasting in BALB/c mice injected with C26 adenocarcinoma cells. ( a–e ) Injection of mice with 20 μg kg −1 PatA 6 days post-injection of C26 adenocarinoma cells prevents muscle wasting without affecting tumour growth. Mice were treated with or without 20 μg kg −1 of PatA starting at 6 days post-injection of C26 cells and every second day thereafter. Mice were subsequently killed 19 days after the injection of C26 cells. ( a ) Photographs of the tumours are representative of n =3 mice per sample group. Bars, 5 mm. Tumour volume ( b ) and weight ( c )±s.e.m. were measured for 3 mice per group. NS refers to non-significance. ( d ) Photograph and ( e ) weight of gastrocnemius muscles isolated from mice described above. Photographs in d are representative of n =3 mice, Bars, 5 mm. Weights in e are presented±s.e.m. from n =3 mice per group. * P <0.05, ** P <0.01 (Student's t -test). ( f–j ) Injection of 20 μg kg −1 PatA in C26 tumour-bearing mice prevents muscle atrophy. ( f ) Effect of 20 μg kg −1 PatA or 50 mg kg −1 AMG on the growth of C26 tumours. Tumour volumes were calculated over a 3-week period. PatA or AMG was only injected into mice on day 13 (indicated on graph by a black arrow) when tumours became palpable and every second day thereafter. The mice were killed on day 22 after the injection of C26 cells. Volumes are presented as ±s.e.m. from n =3 mice. ( g ) Weight of tumours and ( h ) gastrocnemius muscles isolated from mice 22 days post-C26 injection treated or not with 20 μg kg −1 of PatA or 50 mg kg −1 AMG, as described above. Weights are presented ±s.e.m. from n =3 mice per group. ( h ) * P <0.05 (Student's t -test). ( i ) Immunohistochemical staining of gastrocnemius muscle fibres isolated from saline as well as C26 tumour-bearing mice treated with or without PatA, as described above. Bars, 20 μm. ( j ) The cross-sectional area of muscle fibres described in i are represented as a frequency histogram from n =2 mice. The mean cross-sectional area of the fibres is indicated in the histogram±s.e.m. Full size image Next, we assessed whether this low dose of PatA could have the same effect on muscle wasting when administered at a stage where the C26-tumour is fully formed. We injected 20 μg kg −1 PatA intraperitoneally into mice, 13 days post-injection of C26 cells. Although, at this time point, body-weight loss was minimum, these mice developed palpable tumours (~300 mm 3 ) and demonstrated a significant decrease in the mass of the gastrocnemius muscle ( Fig. 3f , Supplementary Fig. S4 ). Under these conditions, PatA, and to a lesser extent AMG, prevented the C26-tumour-induced loss of the gastrocnemius muscles without affecting tumour growth and mass ( Fig. 3f–h ). In addition, PatA also prevented the loss of the quadriceps muscle and rescued, by ~20%, the mean cross-sectional area of both the gastrocnemius and quadricep muscle fibres ( Fig. 3i,j ; Supplementary Fig. S5 ). Interestingly, our data show that these effects were not due to a decrease in IL-6 secretion ( Supplementary Fig. S6 ). Together, these data demonstrate that a low dose of PatA is sufficient to prevent in vivo cancer-induced muscle wasting, without affecting the tumours themselves. To determine whether PatA is also effective in reversing muscle wasting, triggered by a tumour-free condition, we used a model in which mice are treated with IFNγ and TNFα. These mice undergo muscle loss in a way that mimics the cachectic-diseased state in cancer [5] , [6] , [35] . IFNγ and TNFα with or without PatA were injected intramuscularly every day during a 5-day period. We then assessed muscle weight and size. We observed that treating mice with 7500U of IFNγ and 3 μg of TNFα significantly reduced the size and weight of both the gastrocnemius and soleus muscles when compared with mice treated with saline. The simultaneous injection of 20 μg kg −1 PatA with the cytokines, however, inhibited these effects ( Fig. 4a–f ). Thus, in a tumour-free environment, a low dose of PatA is also able to prevent the onset of muscle wasting in vivo . 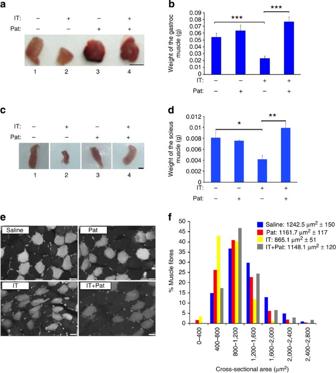Figure 4: PatA prevents the loss of muscle in mice injected intramuscularly with IFNγ/TNFα. (a–d) Effect of PatA on IFNγ/TNFα-treated gastrocnemius and soleus muscles. Photograph (a) and weight (b) of gastrocnemius muscle isolated from mice, 5 days after injection, with or without IFNγ and TNFα in the presence or absence of 20 μg kg−1of PatA. Bars ina, 5 mm. Weights inbare plotted±s.e.m. fromn=9 mice. ***P<0.001 (Student'st-test). Photograph (c) and weight (d) of soleus muscle isolated from mice treated, as described above. Bars inc, 1 mm. Weights in d are plotted ±s.e.m. fromn=3 mice. *P<0.05, **P<0.01 (Student'st-test). (e) Immunohistochemical staining was performed, as described inFigure 3,on soleus muscle fibres isolated from mice injected with IFNγ and TNFα in the presence or absence of 20 μg kg−1of PatA. Bars, 20 μm. (f) The cross-sectional area of muscle fibres obtained from the muscles ineare represented as a frequency histogram fromn=3 mice. The mean cross-sectional area of the fibres is indicated in the histrogram±s.e.m. Figure 4: PatA prevents the loss of muscle in mice injected intramuscularly with IFNγ/TNFα. ( a–d ) Effect of PatA on IFNγ/TNFα-treated gastrocnemius and soleus muscles. Photograph ( a ) and weight ( b ) of gastrocnemius muscle isolated from mice, 5 days after injection, with or without IFNγ and TNFα in the presence or absence of 20 μg kg −1 of PatA. Bars in a , 5 mm. Weights in b are plotted±s.e.m. from n =9 mice. *** P <0.001 (Student's t -test). Photograph ( c ) and weight ( d ) of soleus muscle isolated from mice treated, as described above. Bars in c , 1 mm. Weights in d are plotted ±s.e.m. from n =3 mice. * P <0.05, ** P <0.01 (Student's t -test). ( e ) Immunohistochemical staining was performed, as described in Figure 3, on soleus muscle fibres isolated from mice injected with IFNγ and TNFα in the presence or absence of 20 μg kg −1 of PatA. Bars, 20 μm. ( f ) The cross-sectional area of muscle fibres obtained from the muscles in e are represented as a frequency histogram from n =3 mice. The mean cross-sectional area of the fibres is indicated in the histrogram±s.e.m. Full size image PatA prevents iNOS-induced muscle wasting One of the key mediators of muscle wasting is the iNOS/NO pathway [2] . As both C26-tumours ( Supplementary Fig. S2 ) and IFNγ/TNFα [6] induce muscle loss by increasing the expression levels of iNOS, we assessed the impact of PatA on its expression in vivo . We observed that 20 μg kg −1 PatA prevented the loss of Myogenin expression in the gastrocnemius treated with IFNγ and TNFα, as described above, and reduced by >50% the levels of the iNOS protein ( Supplementary Fig. S7a–c ). Northern blot analysis showed that PatA had no effect on the levels of the iNOS mRNA, but it prevented the IFNγ/TNFα-induced loss of the Myogenin and MyoD messages ( Supplementary Fig. S7d–g ). These data clearly indicate that in vivo a low dose of PatA prevents muscle wasting by blocking the expression of pro-cachetic factors, such as iNOS, while rescuing the expression of promyogenic factors, such as MyoD and Myogenin. Next, we delineated the mechanism by which PatA mediates these opposite effects. C2C12 muscle fibres were treated with IFNγ and TNFα in the presence or absence of PatA, as described above ( Fig. 2 ). Consistent with our in vivo data ( Supplementary Fig. S7 ), we observed that 0.1 μM PatA prevented IFNγ/TNFα-induced fibre loss by significantly reducing the expression levels of iNOS protein and NO release while preventing the loss of MyoD and Myogenin mRNAs ( Fig. 5a–g ). The PatA-induced decrease in iNOS expression and NO release was also observed with lower doses of PatA (0.1 to 0.0125 μM) ( Supplementary Fig. S8 ). These data, combined with the fact that PatA did not affect the steady-state level of iNOS mRNA ( Fig. 5d,e ), nor the expression level of IFNγ/TNFα-induced IL-6 (a well-characterized promoter of NF-κB/cancer-induced muscle wasting [1] ) ( Supplementary Fig. S9 ), led us to conclude that PatA inhibits iNOS expression by acting on posttranscriptional events (mRNA stability, cellular movement or translation) and not on NF-κB-induced iNOS transcription. 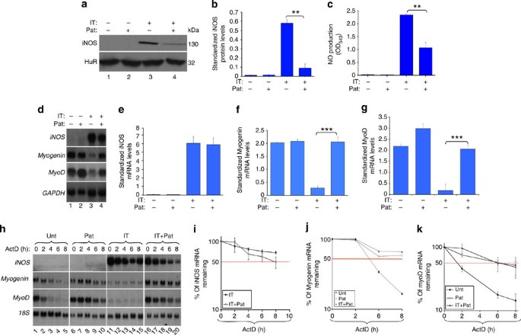Figure 5: PatA differentially regulates the expression of iNOS and MyoD in cytokine-treated myofibres. (a–c) PatA significantly reduces iNOS protein level and NO release. (a) Western blot analysis using an antibody detecting iNOS was performed to determine the effect of (0.1 μM) PatA on iNOS protein expression in cytokine-treated muscle fibres. HuR protein levels are included as loading controls. (b) The iNOS protein levels above were quantified, normalized against the HuR protein levels and plotted ± the s.e.m. from three independent experiments. **P<0.01 (Student'st-test). (c) NO release by C2C12 myofibres was assessed with GRIESS reagent 24 h after treatment with or without PatA in the presence or absence of IFNγ/TNFα, as described above. NO levels are plotted±the s.e.m. from three independent experiments. **P<0.01 (Student'st-test). (d–k) Unlike the MyoD and Myogenin mRNA, the steady-state levels and half-life of the iNOS mRNAs are not affected by PatA. (d) Total mRNA was collected from myofibres treated, as described above, and analysed by northern blot to determine iNOS, MyoD and Myogenin mRNA levels. iNOS (e), Myogenin (f) and MyoD (g) mRNA levels, quantified using the ImageQuant software and standardized against GAPDH mRNA levels, were plotted±the s.e.m. from three independent experiments. (f,g) ***P<0.001 (Student'st-test). (h) The stability of the iNOS, MyoD and Myogenin mRNAs was determined by incubating the above stated fibres with 5 μg ml−1of ActD for the indicated periods of time, and the level of iNOS, MyoD and Myogenin mRNAs was determined by northern blot analysis. The stability of iNOS (i), Myogenin (j) and MyoD (k) mRNAs was quantified, as described above, using the ImageQuant software program. Levels were then standardized against 18S rRNA levels and plotted as the percentage±the s.e.m. of three independent experiments of remaining mRNA compared with message levels at the 0 h time point (where there is a 100% maximum mRNA level). Figure 5: PatA differentially regulates the expression of iNOS and MyoD in cytokine-treated myofibres. ( a–c ) PatA significantly reduces iNOS protein level and NO release. ( a ) Western blot analysis using an antibody detecting iNOS was performed to determine the effect of (0.1 μM) PatA on iNOS protein expression in cytokine-treated muscle fibres. HuR protein levels are included as loading controls. ( b ) The iNOS protein levels above were quantified, normalized against the HuR protein levels and plotted ± the s.e.m. from three independent experiments. ** P <0.01 (Student's t -test). ( c ) NO release by C2C12 myofibres was assessed with GRIESS reagent 24 h after treatment with or without PatA in the presence or absence of IFNγ/TNFα, as described above. NO levels are plotted±the s.e.m. from three independent experiments. ** P <0.01 (Student's t -test). ( d–k ) Unlike the MyoD and Myogenin mRNA, the steady-state levels and half-life of the iNOS mRNAs are not affected by PatA. ( d ) Total mRNA was collected from myofibres treated, as described above, and analysed by northern blot to determine iNOS, MyoD and Myogenin mRNA levels. iNOS ( e ), Myogenin ( f ) and MyoD ( g ) mRNA levels, quantified using the ImageQuant software and standardized against GAPDH mRNA levels, were plotted±the s.e.m. from three independent experiments. ( f , g ) *** P <0.001 (Student's t -test). ( h ) The stability of the iNOS, MyoD and Myogenin mRNAs was determined by incubating the above stated fibres with 5 μg ml −1 of ActD for the indicated periods of time, and the level of iNOS, MyoD and Myogenin mRNAs was determined by northern blot analysis. The stability of iNOS ( i ), Myogenin ( j ) and MyoD ( k ) mRNAs was quantified, as described above, using the ImageQuant software program. Levels were then standardized against 18S rRNA levels and plotted as the percentage±the s.e.m. of three independent experiments of remaining mRNA compared with message levels at the 0 h time point (where there is a 100% maximum mRNA level). Full size image As PatA differentially affected the expression levels of iNOS, MyoD and Myogenin mRNAs, we first assessed its effect on the stability of these messages. Actinomycin D (Act D) pulse-chase experiments [41] showed that the iNOS mRNA was highly expressed with a half-life of greater than 8 h in myofibres exposed to IFNγ/TNFα. The addition of 0.1μM PatA, however, did not affect the half-life of this message ( Fig. 5h,i ). Unfortunately, the low levels of MyoD and Myogenin mRNAs in myofibres exposed to IFNγ/TNFα alone ( Fig. 5d , lane 3 and Fig. 5h ) prevented us from determining the half-life of these messages under these conditions. Interestingly, however, 0.1 μM PatA not only rescued the expression of MyoD and Myogenin mRNAs in IFNγ/TNFα-treated myofibres but also increased their half-lives by >4 h ( Fig. 5d, f–h and j,k ). These observations clearly show that one way by which a low dose of PatA protects muscles from the IFNγ/TNFα-induced loss is by triggering two opposite effects. Indeed, although PatA prevents the expression of procachectic factors such as iNOS, it promotes the expression and the stabilization of mRNAs encoding promyogenic factors such as MyoD and Myogenin. We next assessed the impact of a low dose of PatA on the cellular localization of its target mRNAs. In situ hybridization experiments revealed that, unlike MyoD and Myogenin mRNAs, 0.1 μM PatA promoted the recruitment of the iNOS mRNA to cytoplasmic foci in IFNγ/TNFα-treated muscle cells ( Fig. 6; Supplementary Fig. S10 ). Recently, others and we have shown that PatA induces the formation of cytoplasmic foci, named SGs [23] , [24] . SGs normally form in response to a variety of stresses to recruit and maintain cellular mRNAs in a translationally repressed state [26] . Co-staining experiments showed that the FXR1 protein co-localized with the iNOS mRNA in these granules in muscle cells treated with both PatA and IFNγ/TNFα ( Fig. 6 ). In addition, eIF4A and HuR [24] , [27] , [42] were also recruited to these PatA-induced foci ( Supplementary Figs S11,12 ). As these granules disassemble in response to treatment with the translation elongation inhibitor cycloheximide [43] , a typical behaviour of bona fide SGs [24] , [28] , our data suggest that these entities are indeed PatA-induced SGs. These results also indicate that, by recruiting the iNOS, but not the MyoD and Myogenin mRNAs to SGs, PatA selectively blocks the synthesis of a procachectic factor while allowing the expression of promoters of muscle fibre formation. 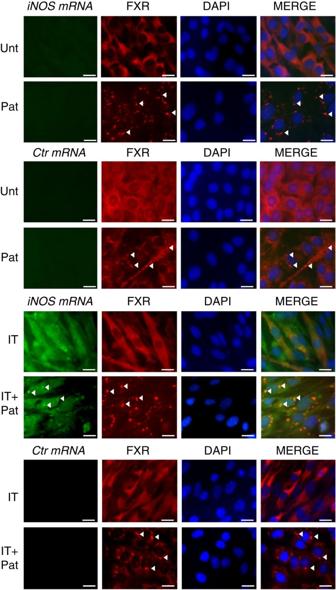Figure 6: The iNOS mRNA is recruited to SGs in IFNγ/TNFα-treated C2C12 cells in the presence of PatA. Differentiated C2C12 myofibres were treated with or without (0.1 μM) PatA in the presence or absence of IFNγ/TNFα. After a period of 24 h, the fibres were fixed, permeabilized and incubated with an anti-sense or sense probe (used as a control probe) to detect iNOS mRNA. DAPI staining and immunostaining against FXR1 were performed to visualize the nucleus and the SGs, respectively. White arrows point to SGs. The results shown are representative of three independent experiments. Bars, 20 μm. Figure 6: The iNOS mRNA is recruited to SGs in IFNγ/TNFα-treated C2C12 cells in the presence of PatA. Differentiated C2C12 myofibres were treated with or without (0.1 μM) PatA in the presence or absence of IFNγ/TNFα. After a period of 24 h, the fibres were fixed, permeabilized and incubated with an anti-sense or sense probe (used as a control probe) to detect iNOS mRNA. DAPI staining and immunostaining against FXR1 were performed to visualize the nucleus and the SGs, respectively. White arrows point to SGs. The results shown are representative of three independent experiments. Bars, 20 μm. Full size image The fact that the iNOS, but not the MyoD or Myogenin mRNAs, is recruited to SGs in response to PatA raised the possibility that, in the presence of PatA, these messages are differentially translated in IFNγ/TNFα-treated muscle fibres. To test this possibility, we followed the effect of PatA on the recruitment of these three mRNAs to polysomes ( Fig. 7a ), a path that is normally taken by all messages undergoing translation [44] . Using sucrose fractionation experiments, we observed that although the iNOS mRNA was recruited to polysomes in IFNγ/TNFα-treated myofibres, this recruitment was reduced by more than twofold with the addition of 0.1 μM PatA. This result is consistent with PatA-induced recruitment of the iNOS mRNA to SGs. In contrast, because MyoD and Myogenin mRNAs did not localize to PatA-induced SGs, their association with polysomes significantly increased when 0.1 μM PatA was added to these cytokines-treated myofibres ( Fig. 7b–c ). The addition of PatA alone to mature myofibres did not, however, affect the association of the MyoD and Myogenin mRNAs with polysomes ( Fig. 7d,e ). We also observed that, similarly to PatA, a low dose of Epi significantly reduced the activation of the iNOS/NO pathway in IFNγ/TNFα myofibres ( Supplementary Fig. S1c,d ). Interestingly, low doses of cycloheximide did not affect the expression of iNOS, nor did it prevent IFNγ/TNFα induced muscle wasting ( Supplementary Fig. S13 ). Therefore, our data demonstrate that low doses of PatA can prevent cachexia by selectively inhibiting the translation of iNOS while promoting the stability and the translation of promyogenic proteins such as MyoD and Myogenin. 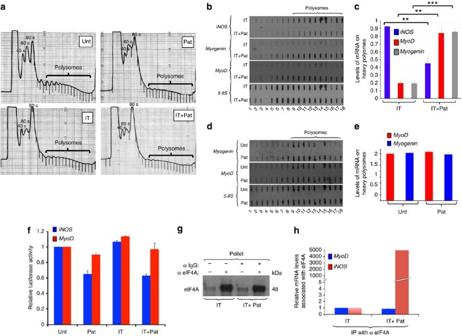Figure 7: PatA differentially affects the translation of iNOS, Myogenin and MyoD mRNAs in cytokine-treated myofibres. (a) Polysome profiles of sucrose fractions obtained from total cell extracts of myofibres treated with or without PatA in the presence or absence of IFNγ/TNFα. (b) The iNOS, Myogenin and MyoD mRNA levels in the fractions, described above, were analysed by slot blot. 5.8S rRNA was included as a loading control. (c) The levels of iNOS, Myogenin and MyoD mRNAs inbwere quantified using the ImageQuant software, standardized against 5.8S mRNA and plotted±the s.e.m. from 3 independent experiments. **P<0.01, ***P<0.001 (Student'st-test). (d,e) MyoD and Myogenin mRNA levels in polysome fractions obtained from untreated and PatA-treated cells were assessed by slot blot (d) and quantified (e), as described above inc. (f) PatA affects the translation of a luciferase reporter containing the iNOS but not the MyoD 5′UTR. Firefly luciferase reporter mRNA containing either the iNOS or MyoD 5′UTR were transfected into muscle cells treated with or without IFNγ/TNFα in the presence or absence of PatA for 24 h. Luciferase activity was subsequently measured, normalized against a co-transfected Renilla luciferase reporter and presented±the s.e.m. of two replicates relative to the untreated samples. (g,h) PatA promotes the association of eIF4A with the iNOS but not the MyoD mRNA. (g) Immunoprecipitations were done using an IgG or an antibody against eIF4A with extracts obtained from myofibres treated for 24 h with IFNγ/TNFα in the presence or absence of PatA. Western blots were then performed to detect eIF4A in the immunoprecipitated pellet. (h) The RNA associated with eIF4A was isolated and analysed by qRT–PCR. Relative levels of both messages associated with eIF4A in IFNγ/TNFα + PatA-treated myofibres are compared with the levels associated with eIF4A in IFNγ/TNFα treated myofibres. Results are presented fromn=1 experiment. Figure 7: PatA differentially affects the translation of iNOS, Myogenin and MyoD mRNAs in cytokine-treated myofibres. ( a ) Polysome profiles of sucrose fractions obtained from total cell extracts of myofibres treated with or without PatA in the presence or absence of IFNγ/TNFα. ( b ) The iNOS, Myogenin and MyoD mRNA levels in the fractions, described above, were analysed by slot blot. 5.8S rRNA was included as a loading control. ( c ) The levels of iNOS, Myogenin and MyoD mRNAs in b were quantified using the ImageQuant software, standardized against 5.8S mRNA and plotted±the s.e.m. from 3 independent experiments. ** P <0.01, *** P <0.001 (Student's t -test). ( d , e ) MyoD and Myogenin mRNA levels in polysome fractions obtained from untreated and PatA-treated cells were assessed by slot blot ( d ) and quantified ( e ), as described above in c . ( f ) PatA affects the translation of a luciferase reporter containing the iNOS but not the MyoD 5′UTR. Firefly luciferase reporter mRNA containing either the iNOS or MyoD 5′UTR were transfected into muscle cells treated with or without IFNγ/TNFα in the presence or absence of PatA for 24 h. Luciferase activity was subsequently measured, normalized against a co-transfected Renilla luciferase reporter and presented±the s.e.m. of two replicates relative to the untreated samples. ( g , h ) PatA promotes the association of eIF4A with the iNOS but not the MyoD mRNA. ( g ) Immunoprecipitations were done using an IgG or an antibody against eIF4A with extracts obtained from myofibres treated for 24 h with IFNγ/TNFα in the presence or absence of PatA. Western blots were then performed to detect eIF4A in the immunoprecipitated pellet. ( h ) The RNA associated with eIF4A was isolated and analysed by qRT–PCR. Relative levels of both messages associated with eIF4A in IFNγ/TNFα + PatA-treated myofibres are compared with the levels associated with eIF4A in IFNγ/TNFα treated myofibres. Results are presented from n =1 experiment. Full size image PatA inhibits iNOS expression in a 5′UTR-dependent manner Recently, small molecules that bind to eIF4A (such as silvestrol and hippuristanol) have been shown to selectively affect the expression of messages by targeting their 5′UTRs [16] , [22] . It is thus conceivable that PatA uses a similar strategy to prevent iNOS expression in muscle fibres undergoing wasting. To test this possibility, we transfected luciferase mRNAs containing the iNOS or the MyoD 5′UTR into myoblasts treated with or without IFNγ/TNFα and assessed, using a luminometer, the effect of PatA on the translation of these two reporter mRNAs. We observed that although PatA decreased the translation of the reporter mRNA containing the iNOS 5′UTR, it did not affect the expression of the reporter construct containing the MyoD 5′UTR ( Fig. 7f ). As PatA has been shown to increase the RNA-binding activity of eIF4A, we next verified whether these opposite effects could be due to a differential association of iNOS and MyoD mRNAs with eIF4A. Immunoprecipitation with eIF4A antibody, in combination with RT–qPCR analysis, showed that although PatA rescued MyoD mRNA expression in IFNγ/TNFα-treated myofibres ( Fig. 5 ), it did not promote its association with eIF4A. However, PatA dramatically increased the association of iNOS mRNA with this translation initiation factor( Fig. 7g,h ). Therefore, these observations, together with the results described in Figs. 6 , indicate that PatA, by acting on the iNOS-5′UTR, promotes the association of the iNOS mRNA with eIF4A and its recruitment to SGs, which in turn inhibits iNOS translation in cytokine-treated myofibres. They also indicate that the inability of PatA to trigger an association between eIF4A and MyoD mRNA and to recruit this message to SGs could be explained by the fact that the MyoD-5′UTR does not respond to PatA. Despite the fact that cachexia-induced muscle wasting has been known for decades as the main cause of death at the late stages of many diseases, the majority of drugs tested so far failed to combat this condition. In this study, we tested the effectiveness of PatA as a potential, new therapeutic drug to prevent muscle wasting induced by either pro-inflammatory cytokines or tumours. We demonstrate that PatA not only prevents TNFα/IFNγ-induced muscle wasting in vitro and in vivo but also interferes with muscle loss triggered by C26-adenocarcinoma tumours. PatA prevents muscle wasting by blocking the expression of the procachetic factor iNOS while rescuing the expression of promyogenic factors MyoD and Myogenin. This differential effect is due to the fact that PatA, by selectively acting on the iNOS-5′UTR, promotes the association of the iNOS mRNA with eIF4A and its recruitment to SGs, where it remains in a translationally repressed state. Conversely, in response to PatA, the MyoD and Myogenin mRNAs are not recruited to SGs but rather associate with heavy polysomes, which leads to the rescue of their expression. As, unlike the iNOS-5′UTR, the MyoD-5′UTR does not respond to PatA, we concluded that the selective effect of PatA depends on the 5′UTRs of target mRNAs. Therefore, our data support a model whereby SGs represent a novel protective mechanism through which compounds such as PatA inhibit the iNOS/NO pathway, which is one of the main promoters of muscle wasting. Likewise, these compounds, by upregulating MyoD and Myogenin expression, not only prevent muscle wasting but may also promote muscle regeneration and maintenance ( Fig. 8 ). 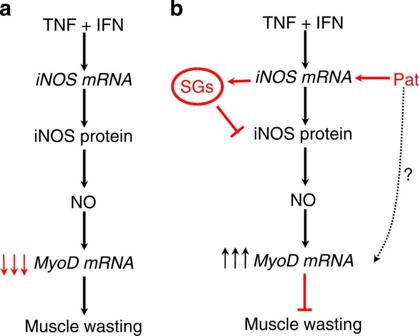Figure 8: Model depicting how PatA prevents cytokine-induced muscle wasting. (a) The cytokines TNFα and IFNγ activate the expression of the iNOS enzyme, which in turn catalyzes NO production. NO then reacts with oxygen radicals, such as superoxide (O2−), forming peroxynitrite, thereby triggering the loss of MyoD expression and muscle wasting6. (b) PatA reverses this outcome by stabilizing and recruiting MyoD mRNA to translationally active polysomes. At the same time, PatA triggers the recruitment of the iNOS mRNA to SGs, blocking its translation. This prevents NO production and the loss of MyoD mRNA. Figure 8: Model depicting how PatA prevents cytokine-induced muscle wasting. ( a ) The cytokines TNFα and IFNγ activate the expression of the iNOS enzyme, which in turn catalyzes NO production. NO then reacts with oxygen radicals, such as superoxide (O 2 − ), forming peroxynitrite, thereby triggering the loss of MyoD expression and muscle wasting [6] . ( b ) PatA reverses this outcome by stabilizing and recruiting MyoD mRNA to translationally active polysomes. At the same time, PatA triggers the recruitment of the iNOS mRNA to SGs, blocking its translation. This prevents NO production and the loss of MyoD mRNA. Full size image The induction of muscle wasting that accompanies many diseases such as cancer and AIDS is due in part to inflammatory mechanisms that promote the loss of MyoD and Myogenin mRNAs, as well as the inhibition of general translation [1] , [5] , [38] , [45] , [46] . We and others have shown that the iNOS/NO pathways is one of main effectors of inflammation-induced muscle wasting. Indeed, the activation of this pathway induces the rapid loss of the MyoD mRNA [6] and also negatively affects general translation by inducing the phosphorylation of eIF2α and inhibiting the mTOR pathway [1] , [38] , [45] , [47] . Our results demonstrate that while elevated doses of PatA, as expected, can inhibit protein synthesis and induce apoptosis in muscle fibres, low doses of this compound, which do not induce apoptosis or affect general translation, prevent muscle wasting by specifically blocking the translation of the iNOS mRNA. PatA, consequently, by targeting this pathway, prevents the negative effect of NO on the expression of promyogenic factors and the inhibition of general translation. The fact that the induction of cachexia involves the inhibition of general translation explains why inhibitors of this process have never been considered as potential anti-cachectic drugs. Therefore, our results showing that an inhibitor of translation initiation, such as PatA, reverses muscle wasting by reestablishing protein translation are novel and unexpected. The eukaryotic initiation factor eIF4A, which functions as a RNA helicase, has been shown to selectively mediate the expression of certain mRNAs by targeting their 5′UTRs [48] , [49] . Recent studies have demonstrated that small molecules such as silvestrol or hippuristanol affect the expression of target mRNAs in a 5′UTR-dependent manner [16] , [22] . Similarly, our results indicate that a low dose PatA inhibits the expression of iNOS but not MyoD by selectively targeting the iNOS 5′UTR. Because silvestrol, hippuristanol and PatA have all been shown to target the function of eIF4A and induce the formation of SGs [16] , [24] ( Supplementary Figs S11,12 ), we concluded that these drugs likely regulate gene expression by recruiting eIF4A-associated mRNAs to SGs, where they are maintained in a translationally inactive state. Therefore, together, our results open the door to design novel strategies to combat the onset of muscle wasting induced by many deadly diseases. Bearing in mind that cachexia is a multifactorial syndrome [1] , to combat its onset and progression, we not only need to block the expression of procachectic factors but also need to activate processes that lead to muscle reconstitution. Because numerous studies have demonstrated the importance of the NF-κB pathway in inducing cachexia [5] , [8] , efforts have been made to test NF-κB inhibitors such as β-hydroxy-β-methylbutyrate and thalidomide as anti-cachectic drugs [1] . Unfortunately, the majority of clinical trials using these type of drugs have not proven to be successful to date [50] . Hence, targeting procachectic factors that act downstream of this pathway, such as iNOS, the expression of which is activated by NF-κB, could be a better therapeutic choice. Small molecules such as PatA seem to be ideal for such a task. At a low dose, PatA not only prevents iNOS-induced muscle wasting but also promotes muscle fibre formation via a novel mechanism that involves the formation of SGs. Given that a low dose of PatA is not toxic for normal muscle fibres, our data demonstrate that PatA, or compounds belonging to the same family, constitute novel tools that alone or in combination with other treatments could be used to combat cahcexia-induced muscle wasting. Cells C2C12 myoblasts (American Type Culture Collection) were grown and induced to differentiate [32] . To trigger their differentiation, C2C12 cells were switched from a media containing 20% fetal bovine serum (Invitrogen) in DMEM (Invitrogen) [32] to a media containing DMEM, 2% horse serum, penicillin/streptomycin antibiotics (Invitrogen), and 50mM HEPES, pH 7.4 (Invitrogen). Myofibres, on the third day following the induction of differentiation, were treated with or without a combination of IFNγ (100 U ml −1 ) and TNFα 20 ng ml −1 ). After a period of 6 h, the myofibres were incubated with or without PatA (concentrations ranging from 0.25 to 0.0125 μM), Cycloheximide (concentrations ranging from 10 to 1 μg ml −1 ) or Episilvestrol (0.05 μM) for 30 min. At this point, the myofibres were washed twice with PBS and re-supplemented with media in the presence or absence of IFNγ/TNFα for the indicated period of time. Reagents and antibodies IFNγ and TNFα were obtained from R&D system. PatA and Episilvestrol [16] , [19] were used as indicated in figure legends. Cycloheximide was obtained from Sigma. The polyclonal (ML13) anti-FXR1 antibody was generously provided by Dr. Edouard Khandjian (Université Laval). Antibodies recognizing both MyHC (MY32; for western blot analysis) and α-tubulin were obtained from Sigma. The anti-iNOS antibody was obtained from BD Biosciences while anti-MyHC (MF-20) and anti-myogenin (F5D) were obtained from Developmental Studies Hybridoma Bank. The anti-caspase 3 cleavage product, anti-phospho-eIF2α, anti-eIF2α, anti-phospho-S6 and anti-S6 antibodies were obtained from Cell Signaling Technology. The anti-eIF4A antibody was from Santa Cruz Biotechnology. Immunoblotting Western blot analyses were performed using total protein extracts and probed with antibodies against HuR [27] (1:10,000), MyHC (1:1,000), tubulin (1:500), iNOS protein (1:10,000), Myogenin (1:250) and eIF4A (1:250). The anti-caspase 3 cleavage product, phospho-eIF2α, eIF2α, phospho-S6 and S6 antibodies were all diluted 1:1,000. Immunofluorescence and in situ hybridization Immunofluorescence experiments were performed as previously described [6] with the following modifications. Briefly, cells were fixed for 30 min with 3% paraformaldehyde, permeabilized with a solution containing 0.1% Triton X-100/phosphate-buffered saline and subsequently incubated with antibodies against HuR [27] (1:1,000), FXR1 (1:1,000) or anti-eIF4A (1:250) (to visualize the formation of stress granules) or myoglobin (1:500) and anti-MyHC (MF-20) (1:1,000) (to verify the integrity of myofibres). On washing, cells were incubated with the appropriately labelled secondary antibody. The proteins were visualized with a Zeiss Axiovision 3.1 microscope (×63 oil objective) and an Axiocam HR (Zeiss) digital camera. For in situ hybridization experiments, C2C12 muscle cells, 1 day post-induction of muscle cell differentiation, were treated with or without IFNγ/TNFα for 24 h in the presence or absence of PatA. The cells were subsequently fixed for 30 min with 3% paraformaldehyde. The iNOS, MyoD and Myogenin mRNAs were then detected by in situ hybridization using primers described in Supplementary methods [25] . De novo protein synthesis The detection of newly synthesized protein was performed [25] , using extracts prepared from cells treated with increasing concentrations of PatA or Cycloheximide for 30 min or with extracts prepared from cells treated with or without IFNγ/TNFα, in the presence or absence of (0.1 μM) PatA, as described above. Muscle fibres were incubated with 35 S-methionine for 30 min to assess de novo protein synthesis. Proteins were resolved by SDS-polyacrylamide gel and stained with Coomassie blue. Quantification of apoptosis Apoptosis was determined by staining myofibres with DAPI to visualize the nucleus. Images corresponding to 10 fields per condition were used to detect the percentage of cells with apoptotic nuclei [51] . Quantification of muscle differentiation and diameter Muscle cell differentiation was determined by quantifying the fusion index of muscle fibres. Fusion index was calculated by determining the number of nuclei in a microscope field in relation to the number of nuclei in myofibres [32] . Measurements of myofibres diameters [52] , taken at two points along their length, were obtained from IF experiments (described above using anti-myoglobin and anti-MyHC antibodies) with fibres treated with or without IFNγ/TNFα in the presence or absence of PatA for 72 h. Detection of NO and IL-6 The release of NO was quantified with using the GRIESS reagent [6] . The secretion of IL-6 was assessed using a commercially available IL-6-specific ELISA kit (eBioscience), as per the manufacturer's instructions. Immunoprecipitation coupled to RT–qPCR Experiments The immunoprecipitation of eIF4A (using an anti-eIF4A from Santa Cruz Biotechnology) and the subsequent extraction and analysis of the RNA by RT–qPCR was performed using total extracts from C2C12 cells and the anti-eF4A antibody, described above [53] . Total RNA from these immunoprecipitates were extracted using TRIZOL. The detection of iNOS and MyoD mRNAs by qPCR was performed using the following primers: iNOS forward primer: 5′-CTTGTGTCAGCCCTCAGAGT-3′, iNOS reverse primer: 5′-GAACTCTTCAAGCACCTCCA-3′, MyoD forward primer: 5′-CGA CAC CGC CTA CTA CAG TG-3′, MyoD reverse primer: 5′-TTC TGT GTC GCT TAG GGA TG-3′. Northern or slot blot and actinomycin D pulse-chase experiments 10 μg of total RNA, extracted from myofibres treated with or without IFNγ/TNFα in the presence or absence of 0.1 μM PatA, were separated on a 1.2% agarose gel containing formaldehyde [6] . Gels were subsequently transferred to nylon membranes and hybridized with labelled cDNA probes detecting iNOS, MyoD, Myogenin and GADPH mRNAs or 18S ribosomal RNA. To analyse the stability of the iNOS, MyoD and Myogenin message, 5 μg ml −1 of Actinomycin D was added to muscle cells for different periods of time, after which cells were collected and total RNA extracted, using TRIZOL [6] . Total RNA was then analysed either by northern or slot blots [25] . Polyribosome fractionation experiments Polyribosome fractions obtained from myofibres treated with or without IFNγ/TNFα for 24 h, in the presence or absence of PatA, were analysed using slot blot [25] . Briefly, myofibres were collected, washed with PBS and centrifuged at 150 g for 5 min. The pellet was resuspended in NWB buffer (20 mM Hepes, pH 7.6, 5 mM MgCl 2 , and 100 mM KCl, 0.5% Nonidet P-40, and Complete protease inhibitors EDTA-free (Roche)) and incubated on ice for 20 min. Cytoplasmic extracts, obtained after the myofibres, were lysed using a Dounce homogenizer, were centrifuged at 130,000 g for 2 h on a sucrose gradient (10–50% w / v ) and then fractionated. RNA was subsequently extracted from the fractions and analysed by slot blot with labelled cDNA probes detecting iNOS, MyoD and Myogenin mRNAs as well as 5.8 rRNA [25] . Luciferase reporter experiments The iNOS and MyoD 5′UTRs were generated by RT–PCR from total RNA isolated from C2C12 myofibres, as described in Supplementary methods . C26-Adenocarcinoma xenograft mouse model Male BALB/c mice (4–6 weeks of age), weighing 20–23 grams were injected subcutaneously with 1×10 6 C26 adenocarcinoma cells [35] . The mice were subsequently injected intraperitoneally 6 days post-C26 injection with or without 20 μg kg −1 or 50 μg kg −1 of PatA. Mice were treated with PatA every second day. The mice were killed by CO 2 inhalation at various periods of time post-C26 injection. Tumour weight and volume were determined at the end of the experiment, and the gastrocnemius muscles were dissected and weighed to assess muscle atrophy. The mice where alternatively injected with 20 μg kg −1 of PatA or 50 mg kg −1 AMG on day 13 post-injection of C26 cells (and every second day thereafter), once tumour growth and muscle loss was physically evident. Tumour growth in C26-injected mice was measured over time using a caliper [54] . Mice were killed by CO 2 inhalation on day 22 post-injection, and the gastrocnemius and quadricep muscles were dissected and used to assess muscle atrophy. These muscles were alternatively frozen, and 8-μm-thick serial sections were stained histochemically for myofibrillar ATPases (pH 10.4), as previously described [55] . Morphometric analyses were then performed on these muscles, using the Aperio ImageScope viewer to determine the cross-sectional area of fibres for each group, n =2 and n =3 mice, respectively, for the gastrocnemius and quadriceps muscles. The dose of PatA used in the experiments described above were determined by assessing the effects of various doses of the drug in these mice, over a 3-week period, and identifying the dose that did not alter physiologically or behaviourally the animals. The animal studies were approved by the McGill University Faculty of Medicine Animal Care Committee. Animals and cytokine treatment The experiments using animal studies were approved by the McGill University Faculty of Medicine Animal Care Committee and comply with guidelines set by the Canadian Council of Animal Care. C57BL/6J mice were injected with saline or 7500 units of IFNγ and 3 μg of TNFα every day for 5 days [6] with or without 20 μg kg −1 of PatA. Mice were sacrificed by CO 2 inhalation 5 day post-injection and the gastrocnemius and soleus muscles were dissected and quick-frozen in liquid nitrogen for future analysis. RNA and protein were subsequently extracted from the gastrocnemius muscles and analysed by slot blot and western blot respectively. The cross-sectional area of the soleus muscle was determined as described above. Statistical analyses Statistical analyses were performed using the Graphpad Prism5 software to determine significance (two tailed, Student's t -test). How to cite this article: Di Marco, S. et al . The translation inhibitor pateamine A prevents cachexia-induced muscle wasting in mice. Nat. Commun. 3:896 doi: 10.1038/ncomms1899 (2012).